Transition-metal-free synthesis of pyrimidines from lignin β-O-4 segments via a one-pot multi-component reaction Heteroatom-participated lignin depolymerization for heterocyclic aromatic compounds production is of great importance to expanding the product portfolio and meeting value-added biorefinery demand, but it is also particularly challenging. In this work, the synthesis of pyrimidines from lignin β-O-4 model compounds, the most abundant segment in lignin, mediated by NaOH through a one-pot multi-component cascade reaction is reported. Mechanism study suggests that the transformation starts by NaOH-induced deprotonation of Cα-H bond in β-O-4 model compounds, and involves highly coupled sequential cleavage of C-O bonds, alcohol dehydrogenation, aldol condensation, and dehydrogenative aromatization. This strategy features transition-metal free catalysis, a sustainable universal approach, no need of external oxidant/reductant, and an efficient one-pot process, thus providing an unprecedented opportunity for N-containing aromatic heterocyclic compounds synthesis from biorenewable feedstock. With this protocol, an important marine alkaloid meridianin derivative can be synthesized, emphasizing the application feasibility in pharmaceutical synthesis. The depletion of fossil resources and rising environmental concerns have led to great interest in biomass utilization [1] , [2] . Lignin, one of the three major components of lignocellulose, has received unique attention because it is regarded as a promising renewable source for aromatic chemicals [3] , [4] , [5] , [6] . So far, numerous efforts have been dedicated to controllable cleavage of the C-O and C-C bonds in lignin to obtain low molecular weight aromatics through introducing hydrogen or oxygen [1] , [7] , [8] . More recently, introducing heteroatom such as nitrogen during lignin depolymerization leading to heteroatom-containing aromatics received much attention, as it is of great potential to expand the product portfolio and to improve the economics of lignin conversion. Importantly, N-heterocyclic aromatic compounds represent a class of vital precursors to pharmaceuticals, dyes and hydrogen storage materials [9] , [10] , [11] ; therefore, production of lignin-derived N-containing aromatics may offer sustainable routes for those value-added compounds. State-of-the-art N-participated lignin conversion is limited to the production of N-containing chemicals from lignin-derived monomers or modified dimer model compounds (Fig. 1 ) [12] , [13] , [14] , [15] , [16] , [17] , [18] , [19] , [20] , [21] , [22] . For instance, hydrogenolysis or oxidation of lignin β-O-4 model compounds catalyzed by transition metals affords monophenols for subsequent amination processes using organic or inorganic N-sources via one or multiple steps to produce different N-containing compounds (Routes 1–3 in Fig. 1 ). In another case, oxidative modification of lignin β-O-4 dimers to ketone derivatives in the presence of oxidant agents such as DDQ (2,3-dichloro-5,6-dicyano-1,4-benzoquinone) [23] and TEMPO (2,2,6,6-tetramethyl-1-piperidyloxy) [24] , followed by different amination processes has also been reported to generate N-containing aromatics (Routes 4–6 in Fig. 1 ). In brief, routes developed so far for the conversion of β-O-4 model compounds, the most abundant segments in lignin, involve hydrogenolysis or oxidative pretreatment. External oxidant or reductant species are essential in such multi-step processes. Moreover, most products are mono-nitrogen-containing aromatics. Our recent progress achieves the synthesis of benzylamines from β-O-4 model compounds, and the feasibility of the production of benzylamines from lignin has also been demonstrated by a two-step process [25] . To the best of our knowledge, no literature reports the direct conversion of β-O-4 model compounds to aromatic heterocyclic compounds containing multiple nitrogen atoms in the absence of transition metal catalysts and external redox reagents, due to the extremely complicated reaction path, and the incompatible catalysis for C-O bond cleavage, C-N formation, and aromatic nitrogen-heterocyclic ring construction. Fig. 1: Production of N-containing aromatics from lignin β-O-4 model compounds. a Amination of monophenols after hydrogenolysis of phenolic β-O-4 model compounds; b conversion of modified β-O-4 model compound to produce N-containing aromatics; c direct conversion of β-O-4 model compound without transition-metals to produce pyrimidines. Full size image Pyrimidines are one type of such N-containing heterocyclic compounds that exhibit broad biological (such as antibacterial, antiallergic, anti-HIV, and antitumor) activities [26] , and have been widely used to design new physiologically and pharmacologically active compounds [27] . Hence, assembling a pyrimidine core has driven considerable investigations. Extensive studies have focused on amidine reactions with coupling partners such as 1,3-dicarbonyl derivatives, α,β-unsaturated ketones, alkynones, 1,2,3-triazines [28] , and alcohols in the presence of organometallic catalysts based on Ir [29] , Ru [30] , Re [31] , Mn [32] , [33] , and Ni [34] . However, most of the methods described so far suffer from employing transition metal catalysts and additives, with complicated ligands, and using non-renewable substrates. On account of the functionalized aromatic scaffold of pyrimidines in structure, the abundant renewable lignin resources would serve as excellent, carbon-neutral starting materials for the development of sustainable routes to pyrimidines, which would also be promising to achieve the green chemistry demand to the environment. In this work, based on the above-listed points, the development of a robust methodology for one-pot pyrimidines synthesis from lignin β-O-4 model compounds is described (Fig. 1 ). The described route is mediated by NaOH in the absence of either transition-metal catalysts or external oxidants/reductants. It combines highly coupled multi-step reactions, including selective C-O bond breaking, aldol condensation, C-C/C-N bond formation, and dehydrogenative aromatization. Thus, it provides an opportunity to prepare pyrimidines from renewable feedstock, which may promote further efforts to explore the abundant lignin resources for the construction of N-containing aromatic heterocyclic compounds. Development of the reaction Lignin β-O-4 linkages represent a predominant portion of all linkages between the primary units. Successful breaking β-O-4 units in model compounds should offer guidance for the depolymerization of realistic lignin. Thus, a typical lignin β-O-4 model compound 1a , accompanied by benzamidine hydrochloride ( 2a ) and benzyl alcohol ( 3a ) has been initially employed to synthesize 2,4,6-triphenylpyrimidine 4a (Fig. 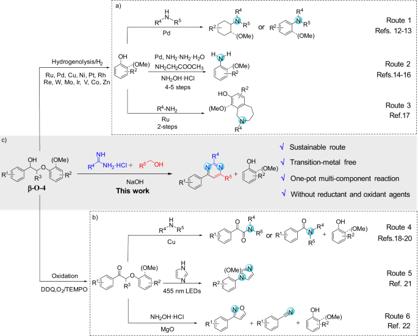Fig. 1: Production of N-containing aromatics from lignin β-O-4 model compounds. aAmination of monophenols after hydrogenolysis of phenolic β-O-4 model compounds;bconversion of modified β-O-4 model compound to produce N-containing aromatics;cdirect conversion of β-O-4 model compound without transition-metals to produce pyrimidines. 2 , entry 1, and Supplementary Table 1 ). We found that the presence of a base played a crucial role in this reaction. In the absence of base, the reaction did not occur (Supplementary Table 1 , entry 1). While NaOH was found to be the most efficient base in stark contrast to KOH, sodium tert -butoxide (t-BuOK), Cs 2 CO 3 , and CH 3 CH 2 ONa (Supplementary Table 1 , entries 2–6). After screening the reaction parameters including solvents, base loading, reaction temperature, and time (Supplementary Tables 1 – 3 and Supplementary Fig. 3 ), the optimized condition was identified, leading to 95% gas chromatograph (GC) yield (93% isolated yield) of 4a based on the amount of 2a , along with 99% GC yield (95% isolated yield) of guaiacol 5a (Fig. 2 , entry 1). In this case, 40.4 wt% of 1a is incorporated in 4a formation (for a detailed calculation process, see Supplementary Fig. 2 ). After the reaction, the solvent tert -amyl alcohol can be easily distilled from the reaction mixture for recycling because the boiling point of tert -amyl alcohol (101.8 °C) is much lower than that of all the reactants (e.g., 1a : 398 °C; 2a : 208 °C; 3a : 205 °C) and the products ( 4a : 330 °C; 5a : 205 °C). Moreover, the reaction can be proceeded at a higher substrate concentration (Supplementary Table 1 , entry 16) but the yields of the targeted products decreased due to severer side reactions. Hence, our strategy not only provides access to a pyrimidine product in high isolated yield, but also achieves co-production of isolated guaiacol in excellent yield, which markedly increases the atom economics. Fig. 2: Conversion of different lignin β-O-4 model compounds to pyrimidines. Conditions: 1 (0.4 mmol), 2a (0.2 mmol), 3a (0.4 mmol), NaOH (1.6 mmol), and tert -amyl alcohol (abbreviation: t -AmOH, 4.0 mL) were mixed in the air at 110 °C, reaction time ( t ) = 20 h; unless otherwise specified, the yields of 4 and 5 were calculated based on the amount of 2a and 1 , respectively. a Isolated molar yield; b GC molar yield was determined by GC-FID using mesitylene as an internal standard. Full size image To examine the generality of this protocol, the activity of various lignin β-O-4 model substrates was explored. Substrates with different functional groups on the aryl ring (Fig. 2 ) are found as fragments in different lignins [1] . 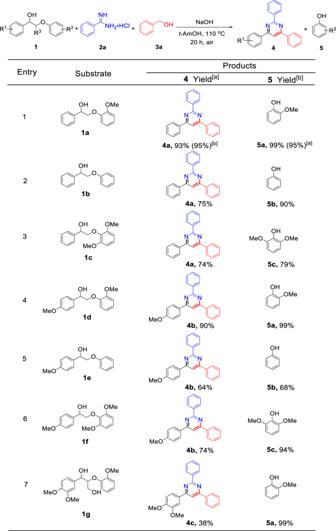Fig. 2: Conversion of different lignin β-O-4 model compounds to pyrimidines. Conditions:1(0.4 mmol),2a(0.2 mmol),3a(0.4 mmol), NaOH (1.6 mmol), andtert-amyl alcohol (abbreviation:t-AmOH, 4.0 mL) were mixed in the air at 110 °C, reaction time (t) = 20 h; unless otherwise specified, the yields of4and5were calculated based on the amount of2aand1, respectively.aIsolated molar yield;bGC molar yield was determined by GC-FID using mesitylene as an internal standard. Under optimized condition, all β-O-4 model compounds were completely consumed to afford the corresponding pyrimidines and monophenols. 2a and 3a reacting with β-O-4 model compounds 1a–1f bearing methoxy groups on both aryl rings afforded moderate to excellent isolated yields of pyrimidine products 4a (74–93%) or 4b (64–90%) along with phenol derivatives 5a – 5c (68–99%) (Fig. 2 , entries 1–6), indicating that the formation of pyrimidine heterocycles occurred associated with selective C-O bond cleavage and C-C/C-N bonds construction in a one-pot fashion. One methoxyl group on the O-terminal aryl ring exhibited a positive influence on the reaction efficiency (90–93%) (Fig. 2 , entries 1 and 4) compared to that bearing no functional group (64–75%) (Fig. 2 , entries 2 and 5) and 2,5-dimethoxy substituents (74%) (Fig. 2 , entries 3 and 6), while methoxyl substitution on the C-terminus aryl ring had little impact on the product yield. Specifically, the highly substituted β-O-4 model compound 1g containing γ-OH functionality was also tolerated, smoothly providing the target product 4c in 38% yield (Fig. 2 , entry 7) despite it has a more complicated structure and contains higher steric hindrance compared to 1a – 1f . Based on the above-described results, it can be concluded that this protocol leads to the successful cleavage of various β-O-4 model compounds and to the synthesis of pyrimidines with good to excellent yields in a one-pot fashion, which thus provides an opportunity for the utilization of lignin to produce value-added N -heterocyclic compounds. This reaction system has proven to be effective not only for a variety of amidine hydrochlorides, but also for a broad range of primary alcohols. As shown in Fig. 3 , eight amidine hydrochlorides 2 have been successfully employed in the transformation, and the yields of corresponding pyrimidine products ( 4d – 4h , 80–94%) from aryl amidine hydrochlorides (Fig. 3 , entries 1–5) were relatively higher than that from aliphatic amidine hydrochloride (Fig. 3 , entry 7, 4j yield 64%). The low yield of pyrimidine 4j is probably due to a negative electronic effect of the ethylamine backbone. Particularly, guanidine hydrochloride also exhibited a high reactivity under standard conditions, giving 4i in 83% yield (Fig. 3 , entry 6). In addition, entries 1–5 in Fig. 3 show that the substituents on the aryl rings of aryl amidine hydrochlorides do not obviously affect the reaction efficiency, regardless of the presence of electron-donating substituents (-CH 3 , -OCH 3 ) or electron-withdrawing substituents (-Cl, -F). A broad range of primary alcohols 3 has also been tested (entries 8–12 in Fig. 3 ). All the reactions proceeded fairly well and yielded 71–92% of pyrimidines 4k – 4o . Notably, two heteroaryl primary alcohols underwent the same reactions to generate high yields of 4n (80%) and 4o (71%), respectively (entries 11–12). Therefore, the above results suggest that such an original protocol for bio-pyrimidines synthesis from lignin β-O-4 segment shows great versatility for all three reaction components. Various lignin model compounds, amidine hydrochlorides, and primary alcohols containing different functional groups are effective in the transformation, representing an interesting breakthrough for the functionalization of lignin products. Fig. 3: Scope of amidine hydrochlorides and primary alcohols. Conditions: 1a (0.4 mmol), 2 (0.2 mmol), 3 (0.4 mmol), NaOH (1.6 mmol), tert -amyl alcohol (abbreviation: t -AmOH, 4.0 mL) were mixed in the air at 110 °C, t = 20 h; the yields of 4 and 5a were calculated based on the amount of 2 and 1a , respectively. a Isolated molar yield; b GC molar yield was determined by GC-FID using mesitylene as an internal standard. Full size image To further determine the compatibility of the reaction system, a β-O-4 polymer mimicking natural lignin was prepared and was used as a substrate for the synthesis of pyrimidine derivative. Though the one-pot, direct conversion of the β-O-4 polymer to pyrimidine was not achieved by reason that the reactive OH group at the para -position of β-O-4 polymer easily reacted with NaOH to produce the sodium phenolate salt under the base environment, an alternative three-step process composed of our key reaction was developed, which achieved 66% overall yield of pyrimidine derivative 4p based on β-O-4 polymer (Supplementary Fig. 1 ). First, binuclear rhodium complex-catalyzed mild depolymerization of β-O-4 polymer led to 4-hydroxyacetophenone (compound I ) in 75% isolated yield, then 4-hydroxyacetophenone reacted with benzyl bromide in the presence of K 2 CO 3 to afford 1-(4-(benzyloxy)phenyl)ethan-1-one (compound II ) in 95% isolated yield, which subsequently reacted with benzamidine hydrochloride and benzyl alcohol, successfully providing pyrimidine derivative 4p in 92% isolated yield (66 wt% yield based on polymer). Mechanistic studies To gain insight into the reaction mechanism, several control experiments were performed to identify possible reaction intermediates. First, treatment of 1a alone under otherwise identical conditions yielded 71% of acetophenone 6 and 82% of guaiacol 5a within 1 h (reaction 1 in Fig. 4a ), indicating that base-catalyzed C-O cleavage of 1a might be the initial reaction step [35] . This assumption was confirmed by the three-component reaction using compounds 6 , 2a , and 3a as substrates (reaction 2 in Fig. 4a ), which afforded a similar yield of 4a (99%) to that in Fig. 2 , entry 1. Hence, in the whole reaction process, NaOH facilitates the cleavage of β-O-4 model compounds to release 6 as an important intermediate for subsequent reactions. Moreover, when benzyl alcohol 3a (Fig. 2 , entry 1) was replaced by benzaldehyde 7 as a substrate, the respective reaction (reaction 3 in Fig. 4a ) also afforded 4a in 82% yield, suggesting that dehydrogenation of 3a into the corresponding aldehyde 7 is another prerequisite step under base condition for the transformation [36] . An additional experiment using 6 , 2a , and 7 as the substrates (reaction 4 in Fig. 4a ) gives a direct evidence by showing that the desired product 4a is obtained in a high yield of 99%. It is well known that a cross-aldol condensation readily occurs between aldehyde and ketone under basic conditions [37] . We therefore assumed that aldol condensation between 6 and 7 would occur to generate chalcone (compound 8 in Fig. 4a ) as an intermediate, which would further react with 2a to form the target product 2,4,6-triphenylpyrimidine 4a . This assumption was supported by another reaction using 8 and 2a as the substrates, which afforded 4a in 59% yield (reaction 5 in Fig. 4a ). On the basis of the above results, a tentative multi-step consecutive pathway can be proposed: the transformation starts with cleavage of the C-O bond in the lignin β-O-4 model compound 1a to release 6 , accompanied by the dehydrogenation of 3a to 7 . Then 6 and 7 undergo a cross-aldol condensation reaction to yield intermediate 8 , which subsequently reacts with 2a to form the six-membered ring intermediate 9 via cyclization reaction. Finally, 9 undergoes an intramolecular dehydrogenative aromatization to furnish 4a (Fig. 4b ). It is worth noting that NaOH plays an important role in each step, viz . selective C-O bond cleavage, cross-aldol condensation, dehydrogenation, and dehydrogenative aromatization, of the whole transformation, and no other catalyst is required, as further supported by the DFT calculation described below. Fig. 4: Mechanistic studies of pyrimidine formation from lignin β-O-4 model compound. a Control experiments and b the proposed pathway. Full size image To obtain insight into the role of NaOH and further disclose the underlying mechanism, DFT calculations have been carried out. Considering that polar solvent tert -amyl alcohol ( t -AmOH) was used and sodium ions exist in the reaction solution, a reaction mediated by sodium hydroxide instead of Zundel anion [38] or hydroxide ion [39] was proposed during DFT calculations (Fig. 5 ). In fact, sodium hydroxide can either deprotonate the C α -H bond along path A or the O-H bond of C α H-OH moiety along path B to form the corresponding intermediates A2 and B2 , respectively, starting from β-O-4 model compound 1a (Fig. 5a ). For C α -H bond cleavage, A2 produces 5a and A4 via a proton transfer step; in the other possible pathway adopting O-H bond cleavage, B2 proceeds a cascade reaction of epoxidation, ring cleavage, and dehydration to form A4 ( B2 → B3 → 5a + B5 → B7 → A4 ), which further tautomerizes into acetophenone 6 catalyzed by base. These calculation results indicate that the C α -H bond and C β -O bond would be broken simultaneously via the transition state ( TS ) TSA1-2 activated by sodium hydroxide (Fig. 5b , path A). The free energy barrier for this C-H/C-O activation step is calculated to be 25.2 kcal/mol. The sodium ion could polarize the β-O atom to lead to a C β -O bond cleavage (paths E and F in Supplementary Fig. 22 ), further illustrating that a sodium ion plays a crucial role in this reaction. Then the proton of the enol moiety of A2 is transferred to the phenol moiety via proton transfer, with a free energy barrier of 3.7 kcal/mol. A3 releases phenol to produce A4 . The proton from the water moiety of A4 is transferred to the enol ion again via TSA4-5 to complete the keto-enol tautomerism with a free energy barrier of 10.2 kcal/mol. Apparently, intermediate 6 can be easily generated along path A, and the C-H activation step is the rate-determining step in the process from β-O-4 model compound 1a to 6 . Compared to path A, the calculated energy barrier of the epoxidation step from B2 to B3 in path B is 29.3 kcal/mol (Fig. 5c , path B), and that for the C-H activation step from B5 to enol A4 is 34.3 kcal/mol. Thus, path A is much more favorable for the C β -O bond cleavage of 1a ( A1 → A2 → 5a + A4 ) than path B ( B1 → B2 → B3 → 5a + B5 → B7 → A4 ). Fig. 5: Computational analysis of the C-O bond cleavage of compound 1a. a Proposed two pathways. b Computational analysis of path A (unit: kcal/mol). c Computational analysis of path B (unit: kcal/mol). Full size image The success of this one-pot, multi-step reaction towards pyrimidines synthesis is governed by two dehydrogenation steps (Figs. 6 and 7 ): benzyl alcohol 3a dehydrogenation to benzaldehyde 7 and dehydrogenative aromatization of 9 to 4a . Fig. 6: The Gibbs free energy profiles for the dehydrogenation of benzyl alcohol 3a. Using O 2 in the air as hydrogen acceptor (path C), acetophenone 6 as hydrogen acceptor (path C-AP), and via hydrogen-acceptor-free pathway (path C-B) (unit: kcal/mol). Full size image Fig. 7: The Gibbs free energy profiles for the dehydrogenation of intermediate 9. Using O 2 in the air as a hydrogen acceptor (path D), acetophenone 6 as a hydrogen acceptor (path D-AP), and via hydrogen-acceptor-free pathway (path D-B) (unit: kcal/mol). Full size image Because the above dehydrogenations are base promoted [40] , it was unclear whether this process employs a hydrogen acceptor or not. Therefore, a control experiment under argon atmosphere was conducted, which resulted in a much lower 4a yield (68%, reaction 6 in Fig. 4a ) compared to that in the air (99%, reaction 2 in Fig. 4a ), illustrating that oxygen in air acted as a hydrogen acceptor in the reaction. It also should be noted that 1-phenylethanol was detected, indicating that intermediate 6 (acetophenone) acted as another hydrogen acceptor. With the aim to verify this speculation and better understand the dehydrogenation mechanism, further DFT calculation was performed. The results, summarized in Fig. 6 , show that benzyl alcohol 3a reacts with sodium hydroxide via TSC1-2 to generate C2 with an energy barrier of 0.2 kcal/mol. In path C using O 2 as the hydrogen acceptor, C2 interacts with O 2 to achieve C3 , followed by the dehydrogenation of C3 . The energy barrier for the dehydrogenation step via TSC3-4 is 10.8 kcal/mol. And in path C-AP using acetophenone 6 as a hydrogen acceptor, the energy barrier of the dehydrogenation via TSC3-4-AP is 17.5 kcal/mol. This is consistent with the experimental observation in reaction 2 Fig. 4a . In addition, the acceptor-free dehydrogenation pathway was also calculated under the same condition, giving two possibilities. As shown in Fig. 6 and Supplementary Fig. 23 , for acceptor-free dehydrogenation, the energy barrier via TSC2-3-B1 would be 34.4 kcal/mol, which is higher than in path C . Moreover, the experiment results further suggest that no hydrogen was detected during the reaction. Combining the DFT calculation and experimental results, it can be concluded that acceptor-free dehydrogenation did not occur for the dehydrogenation of benzyl alcohol. Similarly, the dehydrogenation of intermediate 9 using both O 2 in the air (path D) and 6 (path D-AP) as hydrogen acceptors was also studied. For comparison, an acceptor-free dehydrogenation pathway (path D-B) was also investigated by DFT calculation. As shown in Fig. 7 , 9 first reacts with sodium hydroxide via TSD1-2 to generate D2 . Then D2 follows path D-B to generate pyrimidine 4a in the absence of a hydrogen acceptor with an energy barrier of 30.1 kcal/mol. Alternatively, D2 goes through D3 and D4 to form 4a in the presence of air with a much lower energy barrier of 3.2 kcal/mol, which is lower than that of path D-AP from D3-AP and D4-AP (13.0 kcal/mol), and H 2 is not detected during the reaction. Apparently, the pathway from 9 to 4a is also not an acceptor-free dehydrogenation reaction. The DFT results summarized in Figs. 6 and 7 illustrate that O 2 in the air acts as a hydrogen acceptor for the dehydrogenation of benzyl alcohol 3a to 7 and 9 to 4a . In addition, the by-product NaOOH in path C and path D could oxidize 3a or 9 to release two NaOH molecules (Supplementary Fig. 24 ). Application in synthesis of meridianin derivatives The potential application of this protocol is further highlighted by the preparation of pharmaceutical intermediates, namely meridianin derivatives. Meridianin derivatives are an important class of natural marine alkaloids that display unique bioactivities, such as high antitumor activity, and therefore are widely used in the pharmaceutical industry [41] , [42] . Typically, meridianin derivatives are synthesized either by a multi-step condensation of substituted indoles with guanidines [42] , [43] , [44] , or by a Suzuki coupling reaction between indolyl boronates and halopyrimidines over palladium catalysts [45] . Based on the above-described route for bio-based pyrimidines, here we established an interesting protocol that allows meridianin derivative production, starting from a lignin β-O-4 model compound through a two-step process (Fig. 8 ). First, intermediate 10 was produced in 69% yield upon isolation by treatment of β-O-4 model compound 1d , guanidine hydrochloride 2g with (1-benzyl-1H-indol-3-yl) methanol 3g . Subsequently, debenzylation of 10 with t -BuOK/DMSO under an oxygen atmosphere successfully afforded the meridianin analog 11 in 70% yield (21.5 wt% based on lignin model compound 1d , Supplementary Fig. 2 ). Such a simple methodology does not require any transition-metal catalyst, thus providing a cost-effective alternative to synthesize value-added meridianin derivatives. Fig. 8: Synthesis of a meridianin derivative from lignin β-O-4 model compound. Step one:synthesis of compound 10 from a mixture 1d , 2g and 3g by this protocol; step two: debenzylation of 10 in the presence of t-BuOK/DMSO under an oxygen atmosphere to afford meridianin derivative 11 . Full size image In summary, we have shown an efficient synthesis of functionalized pyrimidines through multi-component reaction of lignin β-O-4 model compounds with amidine hydrochlorides and primary alcohols under transition-metal-free conditions. A highly coupled cascade process, including cleavage of C-O bonds, alcohol dehydrogenation, aldol condensation, and dehydrogenative aromatization reaction has been established to selectively afford a wide range of alkylated and arylated heterocyclic pyrimidines in a one-pot fashion. The methodology can also be applied to assemble meridianin derivatives, which underlines the applicability of this protocol for the synthesis of pharmaceuticals. This protocol paves the way toward applications of lignin, creating a bridge between renewable biomass and pharmaceutical synthesis, and pushes forward one-pot conversion of lignin to value-added pharmaceutical molecules. Further exploration on native lignin is undergoing. Typical procedure for the pyrimidine synthesis from lignin β-O-4 model compound Lignin model compound (0.4 mmol), the primary alcohol (0.4 mmol), benzamidine hydrochloride (0.2 mmol), NaOH (1.6 mmol), internal standard mesitylene (8 mg), and t -AmOH (4 mL) were placed in the pressure tube (35 mL). The mixture was sealed and heated to 110 °C for 20 h. After the reaction, the solution was cooled to room temperature, and ethyl acetate (6 mL) was added to the mixture. Then hydrochloric acid (2 M) was used to acidify the aqueous solution to pH = 1. The organic phase was analyzed by GC-FID to determine the yield of phenol derivatives. Then the solvent was evaporated under reduced pressure, and the crude products were purified by column chromatography using petroleum ether/ethyl acetate (9:1) to obtain the desired products. Details of DFT calculations In this work, ωB97X-D [46] functional was used for the DFT calculation, which considered the dispersion correction. And the Pople-type triple-ζ split-valence basis sets 6–311+G(d,p) are used for the optimization of all structures. The solvation effect of tert -amyl alcohol ( ε = 5.78) was simulated by the SMD [47] continuum solvent mode. The Cartesian coordinates of all optimized structures are given in the Supporting Information. The calculations were performed using Gaussian 09 program [48] . 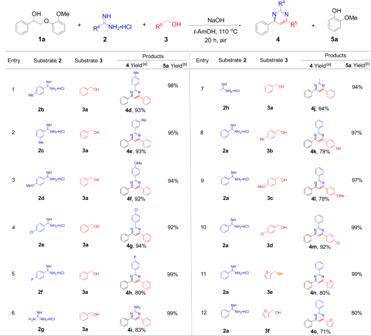Fig. 3: Scope of amidine hydrochlorides and primary alcohols. Conditions:1a(0.4 mmol),2(0.2 mmol),3(0.4 mmol), NaOH (1.6 mmol),tert-amyl alcohol (abbreviation:t-AmOH, 4.0 mL) were mixed in the air at 110 °C,t= 20 h; the yields of4and5awere calculated based on the amount of2and1a, respectively.aIsolated molar yield;bGC molar yield was determined by GC-FID using mesitylene as an internal standard. 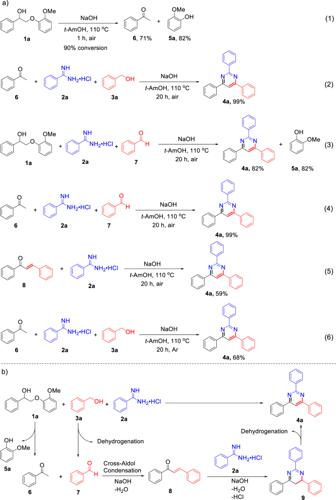Fig. 4: Mechanistic studies of pyrimidine formation from lignin β-O-4 model compound. aControl experiments andbthe proposed pathway. All transition states were confirmed with only one imaginary frequency integrated with intrinsic reaction coordinates [49] calculations. 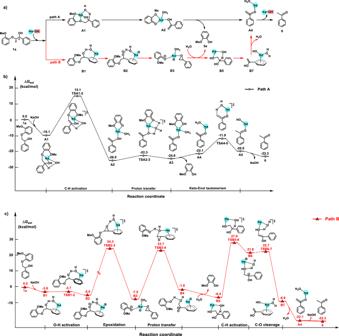Fig. 5: Computational analysis of the C-O bond cleavage of compound 1a. aProposed two pathways.bComputational analysis of path A (unit: kcal/mol).cComputational analysis of path B (unit: kcal/mol). 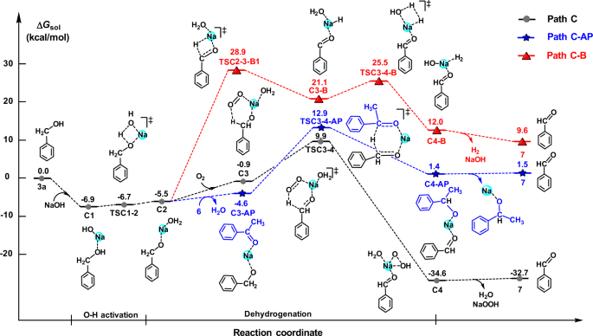Fig. 6: The Gibbs free energy profiles for the dehydrogenation of benzyl alcohol 3a. Using O2in the air as hydrogen acceptor (path C), acetophenone6as hydrogen acceptor (path C-AP), and via hydrogen-acceptor-free pathway (path C-B) (unit: kcal/mol). 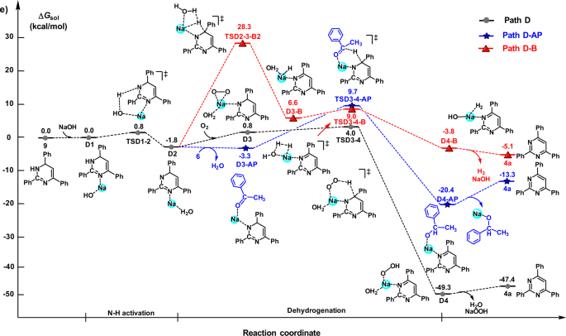Fig. 7: The Gibbs free energy profiles for the dehydrogenation of intermediate 9. Using O2in the air as a hydrogen acceptor (path D), acetophenone6as a hydrogen acceptor (path D-AP), and via hydrogen-acceptor-free pathway (path D-B) (unit: kcal/mol). 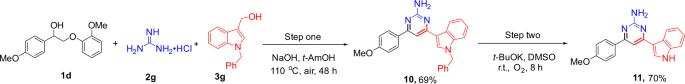Fig. 8: Synthesis of a meridianin derivative from lignin β-O-4 model compound. Step one:synthesis of compound10from a mixture1d,2gand3gby this protocol; step two: debenzylation of10in the presence of t-BuOK/DMSO under an oxygen atmosphere to afford meridianin derivative11. All energies discussed above are Gibbs free energies calculated at 298.15 K. For more information about the DFT calculations, see Supplementary information 1.5 and Supplementary Data 1 – 3 .